Disrupting MLC1 and GlialCAM and ClC-2 interactions in leukodystrophy entails glial chloride channel dysfunction Defects in the astrocytic membrane protein MLC1, the adhesion molecule GlialCAM or the chloride channel ClC-2 underlie human leukoencephalopathies. Whereas GlialCAM binds ClC-2 and MLC1, and modifies ClC-2 currents in vitro , no functional connections between MLC1 and ClC-2 are known. Here we investigate this by generating loss-of-function Glialcam and Mlc1 mouse models manifesting myelin vacuolization. We find that ClC-2 is unnecessary for MLC1 and GlialCAM localization in brain, whereas GlialCAM is important for targeting MLC1 and ClC-2 to specialized glial domains in vivo and for modifying ClC-2’s biophysical properties specifically in oligodendrocytes (OLs), the cells chiefly affected by vacuolization. Unexpectedly, MLC1 is crucial for proper localization of GlialCAM and ClC-2, and for changing ClC-2 currents. Our data unmask an unforeseen functional relationship between MLC1 and ClC-2 in vivo , which is probably mediated by GlialCAM, and suggest that ClC-2 participates in the pathogenesis of megalencephalic leukoencephalopathy with subcortical cysts. Several forms of leukodystrophies, degenerative disorders affecting the white matter of the brain, are associated with vacuolization of myelin sheaths that enwrap axons of central neurons. A particular subentity of this disease, megalencephalic leukoencephalopathy with subcortical cysts (in short MLC), can be caused by mutations in either MLC1 (ref. 1 ), encoding a protein predicted to span the plasma membrane eight times, or less frequently in GLIALCAM [2] , [3] , which encodes the adhesion molecule GlialCAM of the immunoglobulin superfamily [4] . MLC1 and GlialCAM bind each other, and this binding originally suggested GLIALCAM as a candidate gene for MLC [2] . GlialCAM was first identified as being downregulated in hepatic cancer (hence, its original name HepaCAM [5] ), but is predominantly expressed in glial cells [6] . GlialCAM co-localizes with its binding partner MLC1 at astrocytic endfeet contacting blood vessels and at astrocyte–astrocyte contacts [7] . GlialCAM and MLC1 share this localization with the ClC-2 chloride channel [8] . In addition to other symptoms [9] , Clcn2 −/− mice display leukodystrophy [8] , suggesting that ClC-2 deficiency might underlie human leukoencephalopathy. Screens for CLCN2 mutations in leukodystrophy patients were initially negative [8] , [10] , but a recent study identified CLCN2 mutations in a distinct form of leukoencephalopathy [11] . Clinical symptoms of either form of the disease include ataxia and sometimes spasticity. On the basis of a limited number of patients, CLCN2 leukodystrophy differs from MLC in the magnetic resonance imaging pattern of affected brains [11] . By contrast, clinical and magnetic resonance imaging features of patients with the MLC1 disease entity (mutations in MLC1 ) are virtually indistinguishable from those affected by MLC2A ( GLIALCAM mutations on both alleles). The disease is more benign in patients with heterozygous GLIALCAM mutations in dominantly inherited MLC2B [2] . GlialCAM binds not only MLC1 but also ClC-2 (ref. 12 ), a widely expressed Cl − channel activated by hyperpolarization and cell swelling [13] , [14] , [15] . ClC-2 is found in both neurons and glia. GlialCAM directs ClC-2 and MLC1 to cell–cell contacts in heterologous expression. This effect is abolished by several point mutations found in MLC2 patients [3] , [7] , [12] . GlialCAM drastically changes ClC-2 currents in various expression systems by increasing their amplitudes and almost abolishing their inward rectification [12] . It thus appears possible that GlialCAM mutations cause leukodystrophy by mislocalizing ClC-2 and/or by affecting its currents. By contrast, no effects of MLC1 on ClC-2 function, localization or abundance were found [12] , [16] . Thus, it remains unclear why patients with MLC1 mutations have the same symptoms as patients with recessive GLIALCAM mutations, who, based on these cell culture data, would be expected to be more severely affected. Here we investigate the functional network of MLC1, GlialCAM and ClC-2 in vivo, and its role in leukodystrophy, by generating mice that lack MLC1 or GlialCAM proteins ( Mlc1 −/− and Glialcam −/− mice, respectively) and Glialcam dn/dn knockin mice harbouring a dominant point mutation found in patients [2] , [12] . All three mouse lines develop progressive myelin vacuolization in the cerebellum. Loss of GlialCAM changes the localization and abundance of ClC-2 and MLC1, and surprisingly loss of MLC1 changes the localization of ClC-2 and GlialCAM. The linearization and enhancement of ClC-2 currents by GlialCAM that is known from heterologous expression is observed in OLs, but not in Bergmann glia (BG). Hence, GlialCAM-dependent anchoring of ClC-2 to plasma membrane domains is not necessarily coupled with changes in ClC-2 current characteristics. Crosses between different Clcn2 and Glialcam models indicate that the pathology observed with loss of GlialCAM or MLC1 may be partially attributed to a secondary loss of ClC-2 function, but that the loss of either GlialCAM or MLC1 has additional pathogenic effects. Mlc1 and Glialcam mouse models Exons 2 and 3 of the Mlc1 gene were deleted to generate Mlc1 −/− mice ( Supplementary Fig. 1a,b ). Western blots confirmed the absence of the MLC1 protein ( Fig. 1a ). A point mutation was inserted into the mouse Glialcam gene that changes G89 in the first immunoglobulin domain to serine ( Supplementary Fig. 1c–e ). This mutation (G89S) is found in MLC patients with dominant disease [2] . Exons 2–4 were flanked by loxP sites to generate GlialCAM knockout ( Glialcam −/− ) mice by crossing Glialcam G89S,loxP (in the following called Glialcam dn ) mice with deleter mice [17] ( Supplementary Fig. 1c,e ). Glialcam dn messenger RNA was expressed at normal levels in the brain ( Fig. 1b ). Western blots showed that the G89S mutation did not reduce GlialCAM levels ( Fig. 1c,d ) and that GlialCAM, although initially called HepaCAM, lacks significant expression in the liver [6] ( Fig. 1a ). As expected, GlialCAM was absent from Glialcam −/− brain. 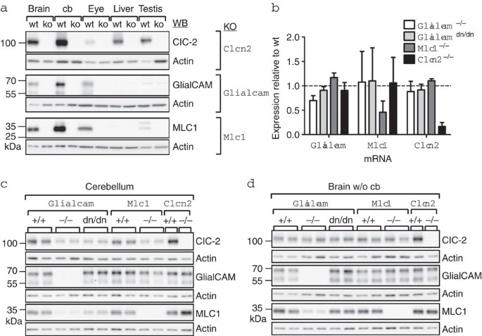Figure 1: Expression of ClC-2, GlialCAM and MLC1 inGlialcamandMlc1mouse models. (a) Western blots for ClC-2 (top), GlialCAM (middle) and MLC1 (bottom) of membrane fractions isolated from organs of WT, andClcn2−/−,Glialcam−/−orMlc1−/−mice, respectively (age: 10–12 weeks). For ClC-2, equal amounts of protein per organ were loaded, whereas for GlialCAM and MLC1 blots, 10 times more protein was loaded for the eye, liver and testis compared with the brain (without cerebellum) and cerebellum (cb). (b) Quantitative real-time PCR to determine levels ofGlialcam,Mlc1andClcn2messenger RNA in the cerebellum of different mouse models. Primers were chosen to amplify regions that were not deleted in corresponding knockout (KO) mice. Bars, relative expression level compared with WT sibling; error bars, s.d. (n≥2). (c) Comparison of ClC-2, GialCAM and MLC1 protein levels in cerebellum and (d) remainder of the brain of WT,Glialcam−/−,Glialcamdn/dn,Mlc1−/−andClcn2−/−mice by western blots of membrane fractions from 10-week-old mice. (c,d) Western blots representative for three independent experiments. Actin served as a loading control. All full size blots can be found inSupplementary Fig. 2. Figure 1: Expression of ClC-2, GlialCAM and MLC1 in Glialcam and Mlc1 mouse models. ( a ) Western blots for ClC-2 (top), GlialCAM (middle) and MLC1 (bottom) of membrane fractions isolated from organs of WT, and Clcn2 −/− , Glialcam −/− or Mlc1 −/− mice, respectively (age: 10–12 weeks). For ClC-2, equal amounts of protein per organ were loaded, whereas for GlialCAM and MLC1 blots, 10 times more protein was loaded for the eye, liver and testis compared with the brain (without cerebellum) and cerebellum (cb). ( b ) Quantitative real-time PCR to determine levels of Glialcam , Mlc1 and Clcn2 messenger RNA in the cerebellum of different mouse models. Primers were chosen to amplify regions that were not deleted in corresponding knockout (KO) mice. Bars, relative expression level compared with WT sibling; error bars, s.d. ( n ≥2). ( c ) Comparison of ClC-2, GialCAM and MLC1 protein levels in cerebellum and ( d ) remainder of the brain of WT, Glialcam −/− , Glialcam dn/dn , Mlc1 −/− and Clcn2 −/− mice by western blots of membrane fractions from 10-week-old mice. ( c , d ) Western blots representative for three independent experiments. Actin served as a loading control. All full size blots can be found in Supplementary Fig. 2 . Full size image Mlc1 −/− , Glialcam −/− and Glialcam dn/dn mice were viable and fertile. Similar to Clcn2 −/− mice [8] , they lacked overt ataxia or spasticity as might have been expected from MLC patients with mutations in the MLC1 or GLIALCAM ( HEPACAM ) genes [1] , [2] . Interdependent protein expression of GlialCAM MLC1 and ClC-2 We wondered whether the expression of ClC-2 and MLC1, both of which bind GlialCAM [2] , [12] , might be changed in the Glialcam mouse models. As myelin vacuolization is most pronounced in the cerebellum of Clcn2 −/− mice [8] and in the present Glialcam and Mlc1 models (see below), we separately studied protein expression in the cerebellum and the rest of the brain. ClC-2 was reduced by ~50% in Glialcam −/− and Glialcam dn/dn cerebella ( Fig. 1c ) but not in the remaining brain ( Fig. 1d ). MLC1 was strongly decreased in the whole brain of Glialcam −/− mice, whereas in Glialcam dn/dn mice, MLC1 was moderately decreased only in the cerebellum ( Fig. 1c,d ). Although MLC1 reportedly binds GlialCAM, but not ClC-2 (refs 2 , 12 ), ClC-2 was reduced in Mlc1 −/− cerebellum ( Fig. 1c ), whereas GlialCAM appeared nearly unchanged ( Fig. 1c,d ). Agreeing with previous work [12] , GlialCAM and MLC1 were not reduced in Clcn2 −/− brain and MLC1 appeared even somewhat increased in Clcn2 −/− cerebellum ( Fig. 1c,d ). Hence, GlialCAM stabilizes MLC1 and the G89S mutant partially retains this stabilizing effect. Both proteins stabilize ClC-2 in the cerebellum. However, ClC-2 is not required for the stability of either GlialCAM or MLC1. These stabilizing effects occur post-transcriptionally as quantitative real-time PCR showed no changes in messenger RNA levels ( Fig. 1b ). Mutually dependent localization of GlialCAM MLC1 and ClC-2 Whereas GlialCAM directs ClC-2 and MLC1 to cell–cell junctions, MLC1 co-transfection does not change the localization of either GlialCAM or ClC-2 (refs 7 , 12 ). We asked whether these in vitro results are relevant in vivo . We first focused on cerebellar BG because their long, straight processes showed particularly prominent, overlapping labelling for ClC-2, MLC1 and GlialCAM ( Fig. 2a ). Moreover, the morphology of BG allows easy visualization of changes in subcellular localization. Whereas ClC-2 disruption had no detectable effect on GlialCAM and MLC1 in BG [12] ( Fig. 2a ), ablation of GlialCAM strongly reduced the labelling for both ClC-2 and MLC1 and changed their localization ( Fig. 2a,b ). Rather than being concentrated along BG processes, both proteins showed faint diffuse staining in the molecular layer and in BG somata where a sizeable portion of immunoreactivity appeared intracellular ( Fig. 2b ). 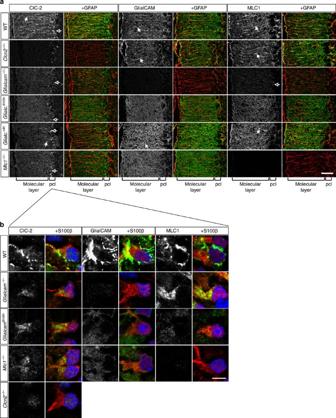Figure 2:GlialcamandMlc1knockout alters localization of ClC-2, GlialCAM and MLC1 in BG. (a) Immunohistochemical (IHC) staining of ClC-2, GlialCAM and MLC1 in the molecular layer of the cerebellum. Co-staining for the astrocytic cytoskeletal protein GFAP (red) visualizes BG processes. Somata of BG are located in the Purkinje cell layer (pcl). Arrows with filled heads point to staining along BG processes, arrows with open heads point to labelled BG somata. Staining respective knockout (KO) sections controls the specificity of antibodies. Note that ClC-2 staining in the Purkinje cell layer ofClcn2−/−mice results from non-specific nuclear staining by the ClC-2 antibody. Scale bar, 50 μm. (b) IHC staining of ClC-2, GlialCAM and MLC1 in BG somata of the cerebellar Purkinje cell layer. Sections were co-stained for the astrocyte marker protein S100β (red) that localizes to the cytoplasm of BG. Nuclei were stained with 4',6-diamidino-2-phenylindole. Scale bar, 5 μm. For each genotype/antibody combination, two brain sections each of at least three different mice were analysed. Figure 2: Glialcam and Mlc1 knockout alters localization of ClC-2, GlialCAM and MLC1 in BG. ( a ) Immunohistochemical (IHC) staining of ClC-2, GlialCAM and MLC1 in the molecular layer of the cerebellum. Co-staining for the astrocytic cytoskeletal protein GFAP (red) visualizes BG processes. Somata of BG are located in the Purkinje cell layer (pcl). Arrows with filled heads point to staining along BG processes, arrows with open heads point to labelled BG somata. Staining respective knockout (KO) sections controls the specificity of antibodies. Note that ClC-2 staining in the Purkinje cell layer of Clcn2 −/− mice results from non-specific nuclear staining by the ClC-2 antibody. Scale bar, 50 μm. ( b ) IHC staining of ClC-2, GlialCAM and MLC1 in BG somata of the cerebellar Purkinje cell layer. Sections were co-stained for the astrocyte marker protein S100β (red) that localizes to the cytoplasm of BG. Nuclei were stained with 4',6-diamidino-2-phenylindole. Scale bar, 5 μm. For each genotype/antibody combination, two brain sections each of at least three different mice were analysed. Full size image In Glialcam dn/dn mice, in which GlialCAM-binding properties might be altered by the G89S mutation in the first extracellular Ig-domain [2] , GlialCAM antibodies did not label the straight BG processes, but still diffusely stained the molecular layer ( Fig. 2a ). Heterozygous Glialcam +/dn mice showed an intermediate phenotype with MLC1 being diffusely labelled in the molecular layer and only small amounts remaining along BG processes ( Fig. 2a ). In both homo- and heterozygous Glialcam dn mice, ClC-2 was retained in BG somata with ClC-2 extending further into BG processes in Glialcam +/dn mice ( Fig. 2a ). Agreeing with the western blot analysis, overall labelling of ClC-2 was reduced in Mlc1 −/− cerebella ( Fig. 2a ), and ClC-2 was retained in BG somata like in Glialcam −/− mice ( Fig. 2a,b ). GlialCAM immunolabelling was similarly diffuse in Mlc1 −/− as in Glialcam dn/dn cerebellum. ClC-2, GlialCAM and MLC1 localization at astrocytic endfeet along blood vessels was reduced in Glialcam −/− , Glialcam dn/dn and Mlc1 −/− mice ( Fig. 3a ). In contrast, the localization of the water channel aquaporin 4 and the K + -channel Kir4.1 (KCNJ10), two proteins reported [18] to reside in a complex with MLC1, were not changed in Mlc1 −/− and Glialcam −/− mice ( Fig. 3b ). 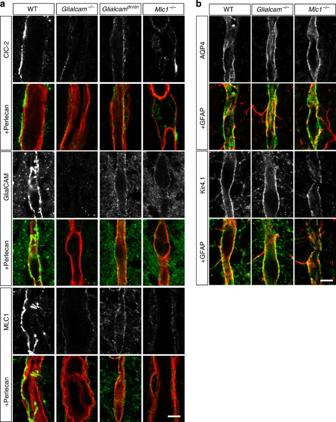Figure 3:GlialcamandMlc1knockout mislocalizes ClC-2, MLC1 and GlialCAM along blood vessels. (a) Immunofluorescent staining of ClC-2, GlialCAM and MLC1 along blood vessels of the hippocampus in mice of different genotypes. Sections were co-stained for perlecan (heparan-sulphate-proteoglycan) a marker for endothelial cells. (b) Immunofluorescent staining of aquaporin-4 (AQP4) and Kir4.1 along blood vessels of the hippocampus. Section were co-stained with the astrocyte marker GFAP that labels astrocytic endfeet contacting blood vessels. Scale bar, 5 μm. For each genotype and antibody combination, two brain sections each of at least two different mice were analysed. Figure 3: Glialcam and Mlc1 knockout mislocalizes ClC-2, MLC1 and GlialCAM along blood vessels. ( a ) Immunofluorescent staining of ClC-2, GlialCAM and MLC1 along blood vessels of the hippocampus in mice of different genotypes. Sections were co-stained for perlecan (heparan-sulphate-proteoglycan) a marker for endothelial cells. ( b ) Immunofluorescent staining of aquaporin-4 (AQP4) and Kir4.1 along blood vessels of the hippocampus. Section were co-stained with the astrocyte marker GFAP that labels astrocytic endfeet contacting blood vessels. Scale bar, 5 μm. For each genotype and antibody combination, two brain sections each of at least two different mice were analysed. Full size image In wild-type (WT) OLs, ClC-2, GlialCAM and MLC1 clustered around their somata ( Fig. 4 ), as previously described for ClC-2 and GlialCAM [8] , [12] . However, unlike ClC-2 and GlialCAM, MLC1 is apparently not expressed in OLs [2] , [19] , [20] . As MLC1 was detected in neighbouring bona fide astrocytes ( Fig. 4 ), the MLC1 staining at oligodendrocytic somata may stem from contact-forming astrocytic processes. 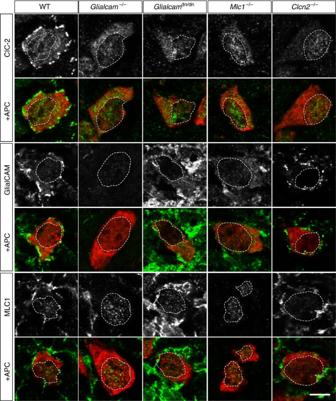Figure 4:GlialcamandMlc1knockout alters the localization of ClC-2, GlialCAM and MLC1 in OLs. Immunohistochemical staining of OLs in fibre tracts of the cerebellum. The cytoplasm of OLs was stained with an antibody against adenomatous polyposis coli (APC) protein. This co-labelling revealed considerable amounts of GlialCAM and MLC1 in cells adjacent to OLs (bona fideastrocytes), as particularly evident inGlialcamdn/dnmice. The faint punctate staining of nuclei with the MLC1 and ClC-2 antibodies is unspecific as revealed byMlc1−/−andClcn2−/−sections, respectively. Note that GlialCAM and MLC1 labelling is unchanged inClcn2−/−mice. Dotted lines mark the location of nuclei within OLs. Scale bar, 5 μm. For each genotype/antibody combination, at least two brain sections each of at least three different mice were analysed. Figure 4: Glialcam and Mlc1 knockout alters the localization of ClC-2, GlialCAM and MLC1 in OLs. Immunohistochemical staining of OLs in fibre tracts of the cerebellum. The cytoplasm of OLs was stained with an antibody against adenomatous polyposis coli (APC) protein. This co-labelling revealed considerable amounts of GlialCAM and MLC1 in cells adjacent to OLs ( bona fide astrocytes), as particularly evident in Glialcam dn/dn mice. The faint punctate staining of nuclei with the MLC1 and ClC-2 antibodies is unspecific as revealed by Mlc1 −/− and Clcn2 −/− sections, respectively. Note that GlialCAM and MLC1 labelling is unchanged in Clcn2 −/− mice. Dotted lines mark the location of nuclei within OLs. Scale bar, 5 μm. For each genotype/antibody combination, at least two brain sections each of at least three different mice were analysed. Full size image In Glialcam −/− , Glialcam dn/dn and Mlc1 −/− mice, ClC-2 no longer formed distinct clusters at the oligodendrocytic plasma membrane but showed faint diffuse, inhomogenous cytoplasmic staining ( Fig. 4 ). Similar changes were seen with G89S-mutant GlialCAM, which was additionally detected in more intense labelling in neighbouring cells. A similar distribution was found with WT GlialCAM in Mlc1 −/− mice. In Glialcam −/− and Glialcam dn/dn mice, MLC1 was diffusely distributed throughout the cytoplasm of adjacent astrocytes, but not in oligodendrocytic somata ( Fig. 4 ). Since OLs lack MLC1, its effect on oligodendrocytic GlialCAM and ClC-2 cannot be cell autonomous. Hence, both GlialCAM and MLC1 were necessary for each other’s correct localization and for the correct targeting of ClC-2 in glial cells, whereas ClC-2 disruption had no significant effect on GlialCAM (see also ref. 12 ) and MLC1 ( Table 1 ). The changed localization of ClC-2 and MLC1 in the Glialcam mouse models is compatible with in vitro results [7] , [12] . However, the effect of MLC1 deletion was unexpected because MLC1 is believed not to bind ClC-2 and to have no role in GlialCAM targeting [7] , [12] . Table 1 Summary of major phenotypes in mouse models of leukodystrophy. Full size table GlialCAM trans -interactions localize MLC1 and ClC-2 in vitro Our in vivo data agree with the effect of GlialCAM on ClC-2 and MLC1 localization in transfected cells, but contrast with the missing impact of MLC1 on GlialCAM [7] , [12] . To systematically analyse the localization of all three proteins, we separately transfected HeLa cells with different combinations of ClC-2, GlialCAM and MLC1 and later combined these cells to form contacts on further growth ( Fig. 5 ). Immunofluorescent labelling revealed that GlialCAM expression in both cells was necessary and sufficient to direct ClC-2 or MLC1 to cell–cell contacts ( Fig. 5a–c , filled arrows). This targeting did not require ClC-2 or MLC1 to be present in both cells ( Fig. 5a,b ). Expression of ClC-2 or MLC1 alone did not affect the localization of GlialCAM, MLC1 or ClC-2 in neighbouring cells even when they co-expressed two of these proteins ( Fig. 5d–g ). Hence, homophilic interactions of GlialCAM in trans may suffice to anchor and concentrate GlialCAM at cell–cell contacts. Binding in cis of GlialCAM to ClC-2 or MLC1 concentrates these latter proteins at the same site without requiring an interaction with ClC-2 or MLC1 on the adjacent cell. 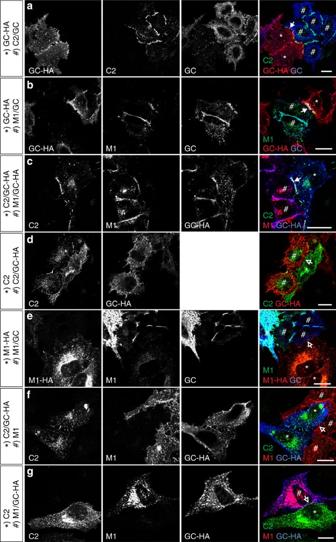Figure 5: Enrichment of ClC-2 GlialCAM and MLC1 at cell–cell contacts requires expression of GlialCAM in both neighbouring cells. HeLa cells were transfected with different combinations ofClcn2,GlialcamandMlc1cDNAs (untagged or haemagglutinin (HA) tagged). Differentially transfected cells were plated onto coverslips and processed for immunofluorescent staining. Individual channel images are displayed in the first three columns, merged images are shown in the fourth column (from left to right). Labels in the lower left corner of each panel indicate the overexpressed protein that was stained with specific antibodies. cDNAs transfected into cells are indicated to the left of each row; in the fourth row cells are labelled with ‘*’ and ‘#’ according to the cDNA combination they were transfected with. Arrows with filled heads point to cell–cell contacts with protein enrichment, arrows with open heads to contacts without protein enrichment. Scale bar, 20 μm; C2=ClC-2; GC=GlialCAM; M1=MLC1. Images shown are representative of at least four images from at least two independent experiments. Figure 5: Enrichment of ClC-2 GlialCAM and MLC1 at cell–cell contacts requires expression of GlialCAM in both neighbouring cells. HeLa cells were transfected with different combinations of Clcn2 , Glialcam and Mlc1 cDNAs (untagged or haemagglutinin (HA) tagged). Differentially transfected cells were plated onto coverslips and processed for immunofluorescent staining. Individual channel images are displayed in the first three columns, merged images are shown in the fourth column (from left to right). Labels in the lower left corner of each panel indicate the overexpressed protein that was stained with specific antibodies. cDNAs transfected into cells are indicated to the left of each row; in the fourth row cells are labelled with ‘*’ and ‘#’ according to the cDNA combination they were transfected with. Arrows with filled heads point to cell–cell contacts with protein enrichment, arrows with open heads to contacts without protein enrichment. Scale bar, 20 μm; C2=ClC-2; GC=GlialCAM; M1=MLC1. Images shown are representative of at least four images from at least two independent experiments. Full size image Modification of ClC-2 currents by GlialCAM and MLC1 in glia When overexpressed in Xenopus oocytes, HEK cells or primary astrocytes, GlialCAM increases ClC-2 currents and almost abolishes its inward rectification [12] . To examine whether these changes occur in vivo , we performed whole-cell patch clamp experiments in brain slices ( Figs 6 and 7 ). Patch pipette solutions contained CsCl to suppress K + currents and the gap junction blocker carbenoxolone to electrically isolate the patched cell from the panglial network [21] . Control experiments with transfected HEK cells confirmed that carbenoxolone did not affect ClC-2 currents ( Supplementary Fig. 3a–c ). Na + currents were suppressed by replacing extracellular Na + with N-methyl-D-glucamine (NMDG + ) ( Supplementary Fig. 3f ). 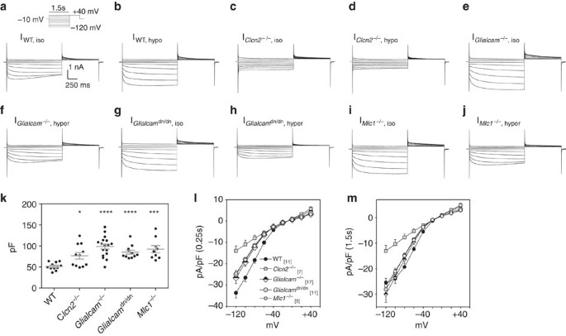Figure 6: ClC-2 currents in BG. (a–j) Current tracings from voltage-clamped BG were averaged for the different mouse models analysed (aged 3–4 weeks). ClC-2 currents were elicited with a voltage pulse protocol. As labelled, measurements were done in either isotonic (iso), hypotonic (hypo) or hypertonic (hyper) bath conditions. Cells were first patched in aCSF and then superfused with an NMDG+-based ‘isotonic’ solution containing carbenoxolone to measure ClC-2 currents. Sometimes, this was followed by superfusion with either a hypotonic or hypertonic bath solution for additional measurements. The number of cells averaged were the following: WT, iso (9); WT, hypo (3);Clcn2−/−, iso (7);Glialcam−/−, iso (15),Glialcam−/−, hyper (5);Mlc1−/−, iso (9);Mlc1−/−, hyper (3),Glialcamdn/dn, iso (11);Glialcamdn/dn, hyper (4). Note that some experiments using shorter and longer pulse protocols were not included for averaging traces shown here but were included for statistical analysis. Traces are scaled uniformly. (k) Individual membrane capacitance values of BG from different genotypes. Horizontal and vertical bars represent mean and s.e.m., respectively.Pvalues between WT and the various mouse models using the Mann–Whitney test: *P≤0.05, ***P≤0.001, ****P≤0.0001. (l,m) Current densities (amplitudes normalized to capacitance) as a function of voltage measured in isotonic bath conditions at 0.25 s (l) or 1.5 s (m) after the beginning of the voltage pulse. Plotted values are mean±s.e.m. The total number of cells in (l,m) is given in panel (l). Legend symbols in (l) apply also to symbols in (m). Figure 6: ClC-2 currents in BG. ( a – j ) Current tracings from voltage-clamped BG were averaged for the different mouse models analysed (aged 3–4 weeks). ClC-2 currents were elicited with a voltage pulse protocol. As labelled, measurements were done in either isotonic (iso), hypotonic (hypo) or hypertonic (hyper) bath conditions. Cells were first patched in aCSF and then superfused with an NMDG + -based ‘isotonic’ solution containing carbenoxolone to measure ClC-2 currents. Sometimes, this was followed by superfusion with either a hypotonic or hypertonic bath solution for additional measurements. The number of cells averaged were the following: WT, iso (9); WT, hypo (3); Clcn2 −/− , iso (7); Glialcam −/− , iso (15), Glialcam −/− , hyper (5); Mlc1 −/− , iso (9); Mlc1 −/− , hyper (3), Glialcam dn/dn , iso (11); Glialcam dn/dn , hyper (4). Note that some experiments using shorter and longer pulse protocols were not included for averaging traces shown here but were included for statistical analysis. Traces are scaled uniformly. ( k ) Individual membrane capacitance values of BG from different genotypes. Horizontal and vertical bars represent mean and s.e.m., respectively. P values between WT and the various mouse models using the Mann–Whitney test: * P ≤0.05, *** P ≤0.001, **** P ≤0.0001. ( l , m ) Current densities (amplitudes normalized to capacitance) as a function of voltage measured in isotonic bath conditions at 0.25 s ( l ) or 1.5 s ( m ) after the beginning of the voltage pulse. Plotted values are mean±s.e.m. The total number of cells in ( l , m ) is given in panel ( l ). Legend symbols in ( l ) apply also to symbols in ( m ). 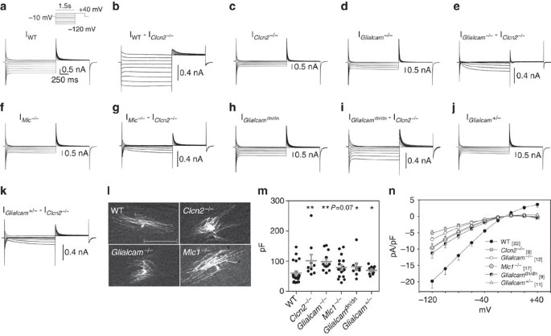Figure 7: ClC-2 currents in OLs. (a,c,d,f,h,j) Current tracings from voltage-clamped OLs of the corpus callosum in isotonic bath solutions were averaged for the different mouse models analysed. Currents were elicited in the same way as described inFig. 5. The number of cells used for averaging traces were WT (22),Clcn2−/−(9),Glialcam−/−(11),Mlc1−/−(17),Glialcamdn/dn(9) andGlialcam+/−(12). (b,e,g,i,k) The average current fromClcn2−/−cells was subtracted from the average current from respective mouse models to obtain the ‘subtracted’ current, which is due to ClC-2 expression. (l) Confocal scans of tissue sections for selected mouse models where OLs were dialyzed with biocytin through the patch pipette. Scale bar, 100 μm. (m) Individual membrane capacitance values of OLs from different genotypes. Horizontal and vertical bars represent mean and s.e.m., respectively. ReportedPvalues were calculated between WT and the various mouse models using the Mann–Whitney test. *P≤0.05, **P≤0.01. (n) Current densities (amplitude normalized to capacitance) measured at the end of a 1.5-s voltage pulse as a function of clamp voltage plotted as mean±s.e.m. Full size image Figure 7: ClC-2 currents in OLs. ( a , c , d , f , h , j ) Current tracings from voltage-clamped OLs of the corpus callosum in isotonic bath solutions were averaged for the different mouse models analysed. Currents were elicited in the same way as described in Fig. 5 . The number of cells used for averaging traces were WT (22), Clcn2 −/− (9), Glialcam −/− (11), Mlc1 −/− (17), Glialcam dn/dn (9) and Glialcam +/− (12). ( b , e , g , i , k ) The average current from Clcn2 −/− cells was subtracted from the average current from respective mouse models to obtain the ‘subtracted’ current, which is due to ClC-2 expression. ( l ) Confocal scans of tissue sections for selected mouse models where OLs were dialyzed with biocytin through the patch pipette. Scale bar, 100 μm. ( m ) Individual membrane capacitance values of OLs from different genotypes. Horizontal and vertical bars represent mean and s.e.m., respectively. Reported P values were calculated between WT and the various mouse models using the Mann–Whitney test. * P ≤0.05, ** P ≤0.01. ( n ) Current densities (amplitude normalized to capacitance) measured at the end of a 1.5-s voltage pulse as a function of clamp voltage plotted as mean±s.e.m. Full size image We first measured BG ( Fig. 6 and Supplementary Fig. 3g–i ) because they prominently express ClC-2, GlialCAM and MLC1 and display strongly changed ClC-2 localization upon disruption of GlialCAM or MLC1 ( Fig. 2a ). We initially identified BG by fluorescence in mice expressing enhanced green fluorescent protein (eGFP) under the control of the glial fibrillary acidic protein (GFAP) promoter [22] and later by dye filling through the patch pipette ( Supplementary Fig. 3d,e ). This labelling revealed no obvious differences in BG morphology among genotypes ( Supplementary Fig. 3e ). Surprisingly, BG Cl − currents did not display the linear current–voltage relationship expected from ClC-2/GlialCAM heteromers [12] ( Supplementary Fig. 3a–c ) but showed the slow activation by hyperpolarization ( Fig. 6a ) that is typical for ClC-2 (without GlialCAM) [14] . Later, an unusual apparent inactivation set in which became faster with hyperpolarization and appeared to reach completion after ~4 s ( Supplementary Fig. 3f ). The absence of these currents from Clcn2 −/− BG ( Fig. 6c ), however, identified them as ClC-2 currents. Whole-cell Cl − currents obtained from BG somata of Glialcam −/− or Glialcam dn/dn mice did not display the expected [12] increased rectification but lacked the apparent inactivation observed in WT glia ( Fig. 6e,g,m , Supplementary Fig. 4a,c,d,f,h,i ). Similar non-inactivating ClC-2 currents were observed with BG from Mlc1 −/− mice ( Fig. 6i,m and Supplementary Fig. 4e,j ). Heterozygous Glialcam +/− BG showed currents similar to WT ( Supplementary Figs 4b,g and 5d ). These results might indicate that, rather than abolishing its rectification as in vitro [12] , in vivo GlialCAM causes ClC-2 to inactivate. However, the cell capacitance of Glialcam −/− , Glialcam dn/dn , Mlc1 −/− and to a lesser extent of Clcn2 −/− BG was increased and more variable compared with WT ( Fig. 6k ). The augmented capacitance suggested an increased cell volume that might change whole-cell currents by reducing the dissipation of Cl − gradients and/or the electrical access to ion channels in distant processes. Indeed, when we superfused BG with hypotonic solution to induce cell swelling (which resulted in the expected increase in cell capacitance ( Supplementary Fig. 5a )), the apparent inactivation of WT and Glialcam +/− Cl − currents was attenuated or even abolished, whereas the non-inactivating currents of Glialcam −/− BG and background currents of Clcn2 −/− BG were unchanged ( Fig. 6b,d and Supplementary Fig. 5b–e ). Conversely, exposure of Glialcam −/− , Glialcam dn/dn or Mlc1 −/− BG to hypertonic solution partially reproduced the current ‘inactivation’ observed in WT BG at isoosmolarity ( Fig. 6f,h,j and Supplementary Fig. 5f–h ). Hence, cell swelling probably contributes to the lack of apparent ClC-2 inactivation in Glialcam −/− and Mlc1 −/− mice. However, cell capacitance and the degree of ‘inactivation’ did not correlate across cells of different genotypes ( Supplementary Fig. 6 ). As WT and mutant BG cells rather segregated into two distinct groups, additional factors like the changed compartmentalization of ClC-2 in mutant mice ( Fig. 2a ) or possibly loss of interaction with other proteins may play a role in suppressing the apparent ‘inactivation’ of ClC-2 currents. The decrease in current amplitudes upon hypertonic shrinkage ( Fig. 6f,h,j ) may be due to reduced electrical accessibility of ClC-2 in cell processes or due to the intrinsic osmosensitivity of ClC-2 (ref. 13 ). From our previous in vitro data [12] we had expected a large decrease of ClC-2 current amplitudes with Glialcam ablation, but averaged current amplitudes of Glialcam −/− BG rather appeared larger than WT ( Fig. 6a,e ). When normalized to cell capacitance, however, current amplitudes of Glialcam −/− , Glialcam dn/dn and Mlc1 −/− BG were moderately smaller compared with WT when measured at early time points ( Fig. 6l ), and nearly unchanged at 1.5 s when WT currents were reduced by the apparent inactivation ( Fig. 6m ). The mild reduction in ClC-2 current density in Glialcam −/− and Mlc1 −/− BG is consistent with the decreased ClC-2 expression in these cells ( Fig. 2 ). Whereas overall BG morphology appears normal in our mouse models, myelin vacuolization (shown below) pointed to pathological changes in OLs, which were therefore included in our analysis ( Fig. 7 and Supplementary Fig. 3j–m ). Their identity was confirmed by dye filling that did not reveal obvious morphological differences among the genotypes ( Fig. 7l ). Unlike BG, Cl − currents of OLs lacked time-dependent activation by hyperpolarization ( Fig. 7a ). About 60% of these currents could be attributed to ClC-2 by comparison with Clcn2 −/− OLs ( Fig. 7a–c and Supplementary Fig. 7a ). Consistent with effects of GlialCAM in heterologous expression [12] , Cl − currents of Glialcam −/− OLs were smaller and displayed the typical activation by hyperpolarization when corrected for background currents of Clcn2 −/− mice ( Fig. 7d,e ). Although currents were small, Cl − currents of Mlc1 −/− and Glialcam +/− OLs appeared similarly rectifying ( Fig. 7f,g,j,k,n and Supplementary Fig. 7b,e ). Currents from Glialcam dn/dn OLs showed less voltage-dependent activation ( Fig. 7h,i and Supplementary Fig. 7d ), consistent with the observation that human mutations in GlialCAM Ig domains interfere with its homophilic binding in trans , but not with its effect on ClC-2 currents [12] . The membrane capacitance of Glialcam −/− , Glialcam dn/dn , Mlc1 −/− and Clcn2 −/− OLs was increased, although not quite to the same extent as in BG ( Fig. 7m compared with Fig. 6k ). Hence, the effect of GlialCAM on ClC-2 currents known from heterologous expression [12] ( Supplementary Fig. 3a–c ) can be observed in OLs, but not in BG ( Table 1 ). On the basis of their increased capacitance, both types of glia appear to be swollen. Leukodystrophy in Glialcam Mlc1 and Clcn2 mouse models Brain sections from Glialcam −/− , Glialcam dn/dn and Mlc1 −/− mice revealed myelin vacuolization that slowly progressed over several months ( Fig. 8a ). Vacuolization was most prominent in fibre tracts of the cerebellum, similar to what was found in Clcn2 −/− mice [8] . While the degree and time course of vacuolization was comparable across Glialcam −/− , Glialcam dn/dn and Mlc1 −/− mice, they altogether developed vacuolization more slowly and less severely than Clcn2 −/− mice. Not until around 1 year of age was discrete vacuolization apparent in cerebellar fibre tracts of Glialcam dn/+ mice. 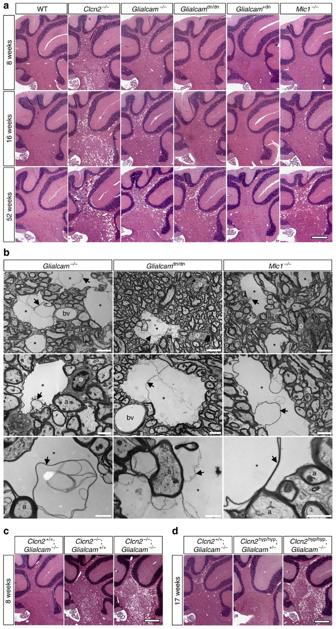Figure 8: Myelin vacuolization inGlialcamandMlc1mouse models. (a) Haematoxylin–eosin (H&E) staining of sagittal paraffin sections of the cerebellum of 8, 16 and 52-week-old mice. (b) Ultrastructural analyses of myelin vacuolization. Myelin vacuolization at different magnifications. asterisk, myelin vacuole; arrow, aberrant myelin sheet inside vacuole; a, axon; bv, blood vessel; o, oligodendrocyte. Scale bars, 5 μm (upper row); 2 μm (middle row); 1 μm (bottom row). (c) H&E staining of the cerebellum of 8-week-oldClcn2−/−,Glialcam−/−double-mutant mice. (d) H&E staining of the cerebellum of 17-week-oldClcn2hyp/hyp,Glialcam−/−double-mutant mice. Scale bar, 400 μm (a,c,d). For each genotype and age, two animals (≥4 sections each) were analysed. Figure 8: Myelin vacuolization in Glialcam and Mlc1 mouse models. ( a ) Haematoxylin–eosin (H&E) staining of sagittal paraffin sections of the cerebellum of 8, 16 and 52-week-old mice. ( b ) Ultrastructural analyses of myelin vacuolization. Myelin vacuolization at different magnifications. asterisk, myelin vacuole; arrow, aberrant myelin sheet inside vacuole; a, axon; bv, blood vessel; o, oligodendrocyte. Scale bars, 5 μm (upper row); 2 μm (middle row); 1 μm (bottom row). ( c ) H&E staining of the cerebellum of 8-week-old Clcn2 −/− , Glialcam −/− double-mutant mice. ( d ) H&E staining of the cerebellum of 17-week-old Clcn2 hyp/hyp , Glialcam −/− double-mutant mice. Scale bar, 400 μm ( a , c , d ). For each genotype and age, two animals (≥4 sections each) were analysed. Full size image After appearing in the cerebellum, vacuolization extends to several brain regions in Clcn2 −/− mice [8] . By contrast, myelin vacuolization was largely restricted to the cerebellum of Glialcam −/− , Glialcam dn/dn and Mlc1 −/− mice even after 1 year ( Supplementary Fig. 8a ). In contrast to early retinal degeneration of Clcn2 −/− mice [9] , the retinae of Mlc1 and Glialcam mouse models were unaffected up to 1 year of age ( Supplementary Fig. 8b ). Electron microscopy revealed vacuoles in myelin sheaths of cerebellar axons from Glialcam −/− , Glialcam dn/dn and Mlc1 −/− mice ( Fig. 8b ). Modest pathological changes were also seen in somata of astrocytes and OLs. Their cytoplasm appeared less electron dense and occasional vacuoles could be observed in astrocytes ( Supplementary Fig. 9 ). One may hypothesize that the leukodystrophy observed in Glialcam −/− and Mlc1 −/− mice might be entirely due to the associated changes in ClC-2 and the resulting consequences for ion homoeostasis [8] . In this case, the additional loss of GlialCAM in Clcn2 −/− / Glialcam −/− mice should not increase the severity of leukodystrophy over that of Clcn2 −/− mice. However, in mice lacking both proteins’ vacuolization appeared earlier and was more severe ( Fig. 8c ). We also crossed Glialcam −/− with Clcn2 hyp/hyp mice that express ClC-2 at <10% of WT levels ( Supplementary Fig. 1f–i ). Clcn2 hyp/hyp mice lacked white matter vacuolization at 17 weeks of age ( Fig. 8d ), demonstrating that a small amount of ClC-2 suffices to maintain myelin integrity as long as ClC-2 is correctly targeted and regulated by GlialCAM. Furthermore, the reduction in ClC-2 protein levels in Glialcam and Mlc1 mouse models is per se not responsible for myelin vacuolization, as their ClC-2 levels are considerably higher than in the hypomorphic mouse. Crossing Clcn2 hyp/hyp with Glialcam −/− mice, however, strongly increased their myelin vacuolization ( Fig. 8d ), suggesting that ClC-2 and GlialCAM operate in the same pathogenic pathway. We have analysed several genetic mouse models for human leukodystrophy to dissect the pathogenic roles of the multipass membrane protein MLC1, the cell adhesion molecule GlialCAM and the Cl − -channel ClC-2. The clustering of these proteins at glial plasma membrane domains depended on the presence of both MLC1 and GlialCAM, but not on ClC-2. The reduction in oligodendrocytic Cl − currents in Glialcam and Mlc1 mouse models indicated that impaired glial ion homoeostasis contributes to MLC disease. Mice lacking both ClC-2 and GlialCAM, however, showed that MLC leukodystrophy cannot be attributed solely to a loss of ClC-2. GlialCAM can bind MLC1 (ref. 2 ) and ClC-2 (ref. 12 ) within the same cell and this binding might be mutually exclusive [12] . GlialCAM also forms cis -homo-oligomers within the membrane [4] , [7] . Homo-oligomer formation does not require the cytoplasmic carboxy terminus [4] , but the relevant binding sites are not yet known. GlialCAM also interacts with itself in trans through its extracellular Ig domains. These domains might interact also with other proteins. Indeed, GlialCAM overexpression increases adhesion to the extracellular matrix and modulates cell migration, and GlialCAM localizes to cell protrusions in spread cells [4] , [23] , [24] . By accumulating at cell–cell contacts through homophilic interactions in trans , GlialCAM targets ClC-2 and MLC1 to these sites in cultured cells [2] , [12] , [25] and stabilizes MLC1 (ref. 25) [25] . By contrast, ClC-2 levels do not increase with GlialCAM co-transfection [12] , and MLC1 expression lacks discernible effects on either GlialCAM [7] or ClC-2 (refs 12 , 16 ). The present systematic analysis of cell pairs revealed that accumulation of ClC-2 or MLC1 at cell–cell junctions only required GlialCAM, but neither ClC-2 nor MLC1, to be present in both cells. Our work demonstrates that GlialCAM localizes ClC-2 and MLC1 to distinct sites also in vivo . Without GlialCAM, MLC1 and ClC-2 accumulated in BG somata. We were surprised that disruption of MLC1 also mislocalized GlialCAM and ClC-2. As MLC1 may not bind ClC-2 (refs 12 , 16 ), its effect on ClC-2 might be mediated by the mislocalization of GlialCAM. However, the effect of MLC1 on GlialCAM is equally unexpected since knockdown of MLC1 in astrocytes changed neither the expression nor the localization of GlialCAM [7] . Does MLC1 stabilize the GialCAM–GlialCAM interaction in vivo , an effect easily overlooked in vitro because of overexpression? Or does MLC1 serve as a co-receptor for GlialCAM, with GlialCAM/MLC1 binding in trans not only to GlialCAM but also to other proteins present in the brain but absent in cell culture? Surprisingly, Mlc1 disruption also destabilized GlialCAM and ClC-2 in OLs, although they apparently lack MLC1 (refs 2 , 19 , 20 ). MLC1 expression appears to be restricted to astrocytes since Mlc1 −/− mice now revealed that previously reported axonal labelling for MLC1 (refs 20 , 26 ) was unspecific. ClC-2, GlialCAM and MLC1 cluster at oligodendrocytic somata close to Cx47 (refs 8 , 12 ), which forms gap junctions with astrocytes [27] . We speculate that astrocytic GlialCAM might be unstable without astrocytic MLC1, which in turn may destabilize the ClC-2/GlialCAM complexes on OLs because they now lack their cognate interaction partner. The G89S mutation introduced into Glialcam dn mice is found in patients with dominantly inherited MLC2B disease [2] . It changes a residue in the extracellular Ig-like domain and probably interferes with binding to ligands. Indeed, when GlialCAM carries disease-causing mutations in Ig domains (for example, G89D that affects the same residue as G89S), neither GlialCAM nor MLC1 or ClC-2 accumulate at cell–cell junctions [2] , [12] . However, mutants like G89D can still bind MLC1 (ref. 7 ) or ClC-2 and can modify its Cl − currents [12] . Similarly, the GlialCAM G89S mutant was mislocalized in Glialcam dn/dn mice in vivo and consequently failed to correctly localize ClC-2 and MLC1. MLC1 abundance was robustly decreased in Glialcam −/− mice, suggesting an increased stability of GlialCAM/MLC1 complexes. The GlialCAM mutant, although mislocalized, partially retained its stabilizing effect on MLC1, in particular outside the cerebellum ( Fig. 1c,d ). No such stabilization was observed for ClC-2, possibly indicating that mutant GlialCAM binds ClC-2 less strongly than MLC1. Western blots suggested that ClC-2 is more efficiently stabilized by GlialCAM in the cerebellum than in the rest of the brain. However, ClC-2 is also expressed in neurons where its expression should not depend on GlialCAM. Hence, this result may be due to a higher glial versus neuronal ClC-2 expression in the cerebellum. ClC-2 is a widely expressed plasma membrane Cl − channel that slowly activates on hyperpolarization, cell swelling and moderately acidic extracellular pH [13] , [15] . These characteristics were observed in heterologous overexpression and in native cells [9] , [28] including neurons [29] , [30] and astrocytes [31] , [32] , [33] . Upon heterologous co-expression, GlialCAM increases ClC-2 currents and drastically changes their properties from inwardly rectifying to a nearly ohmic current–voltage relationship, an effect that does not require GlialCAM–GlialCAM trans -interactions [12] . It has remained unclear whether the linearization of ClC-2 currents also occurs in vivo or results from non-physiological overexpression. Indeed, other groups have shown that native astrocytes display typical hyperpolarization-activated ClC-2 currents [31] , [32] , [33] , [34] . Strikingly, we observed the expected effect of GlialCAM on Cl − currents only in OLs, although BG also co-expresses ClC-2 and GlialCAM. Glialcam −/− OLs displayed typical inwardly rectifying ClC-2 currents, whereas similarly background corrected currents from WT cells were larger and neither showed time dependence nor inward rectification. In contrast to OLs, BG showed hyperpolarization-activated Cl − currents with or without GlialCAM. Current amplitudes at Glialcam −/− or Mlc1 −/− BG somata were moderately increased, but when normalized to membrane capacitance they were rather decreased. Cell swelling, as indicated by increased membrane capacitance of Glialcam −/− or Mlc1 −/− BG, may have improved the electrical accessibility of BG processes that retain some ClC-2. Indeed, current amplitudes were reduced when Glialcam −/− , Glialcam dn/dn and Mlc1 −/− BG were shrunk by exposure to hypertonicity. Why did GlialCAM change the rectification of ClC-2 in OLs, but neither at BG somata nor in astrocytes [31] , [32] , [33] , [34] if all three cell types co-express these two proteins? One may hypothesize that MLC1, which is expressed in BG but not in OLs, may interfere with the biophysical effect of GlialCAM on ClC-2 currents. However, the additional expression of MLC1 did not change the effect of GlialCAM on ClC-2 currents in Xenopus oocytes [12] . An easy explanation would be a higher GlialCAM/ClC-2 ratio in OLs, an assumption difficult to verify by immunohistochemistry. Bolstering this notion, overexpression of GlialCAM in native astrocytes increased Cl − currents and reduced their rectification [12] . However, the strong effect of GlialCAM on ClC-2 localization and abundance in BG suggests that the majority of ClC-2 is normally anchored and stabilized by GlialCAM. This anchoring might require less GlialCAM per ClC-2 than the change in channel rectification. The stoichiometry of ClC-2/GlialCAM binding is currently unknown. One could speculate that binding of one GlialCAM molecule to a homodimeric ClC-2 channel suffices for anchoring, but that two (or more) GlialCAM β-subunits are required to change the gating of the two ClC-2 pores [35] . An increase of up to twofold in membrane capacitance of BG and OLs suggested that their volume was increased when either MLC1, GlialCAM or ClC-2 was lacking. Independent evidence for cell swelling was obtained from the apparent inactivation of ClC-2 currents in WT BG that could be reversed by hypo-osmotic swelling and was abolished in Glialcam −/− cells. A common denominator for the increase in glial cell volume may be a reduction of ClC-2 currents. Loss of ClC-2, which is swelling activated [13] , [15] and constitutively open when modified by GlialCAM [12] may cause cell swelling because the Cl − equilibrium potential of glia [36] , [37] , [38] predicts an outwards direction of Cl − flux and associated water transport. Although ClC-2 currents at BG somata were not reduced in Glialcam or Mlc1 mouse models, ClC-2 was strongly decreased along BG processes. At these sites, which escape our patch clamp analysis, ClC-2 currents might be linearized and enhanced by GlialCAM and might influence cell volume. MLC1 was reported [39] to stimulate the ubiquitous volume-regulated anion channel (VRAC) that is distinct from ClC-2 (ref. 13 ) and is not known at the molecular level [40] . Short interfering RNA-mediated knockdown of GlialCAM or MLC1 reduced VRAC currents [25] . This effect is probably indirect as AQP4 knockdown also reduced astrocytic VRAC currents [41] . Since both ClC-2 and VRAC mediate Cl − currents, and because membrane capacitance was also increased in Clcn2 −/− mice, the simplest explanation for glial swelling remains a lack of ClC-2. Another factor may be the lack or downregulation of GlialCAM-mediated adhesion in Glialcam and Mlc1 mouse models, respectively. The somewhat larger increase in cell capacitance of BG from Glialcam −/− and Mlc1 −/− mice compared with Clcn2 −/− mice is compatible with this notion. Disruption of all three genes, that is, Clcn2 , Glialcam and Mlc1 , entails leukodystrophy in mice and humans. Since GlialCAM binds to both ClC-2 and MLC1 and disruption of either Glialcam or Mlc1 affects the localization and abundance of the two other proteins, this raises the question whether loss-of-function mutations in those genes cause leukodystrophy through a common pathway. Four observations suggest loss of ClC-2 function as the prime suspect for such a pathway: first, ClC-2 localization was changed upon Glialcam or Mlc1 disruption, whereas lack of ClC-2 had no detectable effect on either GlialCAM or MLC1. Second, OLs, the cells mainly affected by vacuolization, showed decreased ClC-2 Cl − currents in both Glialcam −/− and Mlc1 −/− mice. As OLs lack MLC1 (refs 2 , 19 , 20 ), the myelin vacuolization in Mlc1 −/− mice may result from the secondary loss of ClC-2 and/or GlialCAM. Third, leukoencephalopathy was more severe in Clcn2 −/− mice than in Glialcam −/− or Mlc1 −/− mice, which retain reduced ClC-2 levels in glia. The fact that disruption of Clcn2 , but not of Glialcam or Mlc1 , additionally causes testicular and retinal degeneration [9] is because of the wider expression pattern of ClC-2 (ref. 14) [14] . Fourth, when Glialcam −/− mice were crossed with Clcn2 hyp/hyp mice that express <10% of WT ClC-2 levels but lack leukodystrophy, myelin vacuolization of resulting Glialcam −/− / Clcn2 hyp/hyp mice was more severe than in Glialcam −/− mice, suggesting a common pathogenic pathway. We have previously hypothesized [8] that ClC-2 disruption causes leukodystrophy by disturbing the buffering of extracellular ions analogous to the postulated role of ClC-2 in regulating the milieu extérieur of sertoli cells and photoreceptors [9] . Indirect support for this model came from the co-localization at astrocytic endfeet of ClC-2 with the K + channel Kir4.1 (refs 42 , 43 ), whose inactivation also entails leukodystrophy [42] , [44] as does ablation of glial connexins 32 and 47 (refs 45 , 46 , 47 ). These proteins are thought to co-operate in ‘K + siphoning’ [48] . This model states that K + released from neurons during action potential repolarization is taken up by Kir4.1 into the connexin-linked astroglial network and is then equilibrated with serum through astrocytic endfeet at blood vessels. Cl − fluxes through ClC-2 may be needed for an overall electroneutral transport across glial plasma membranes during K + siphoning. The linearization of ClC-2 currents by GlialCAM may be important for K + siphoning as a rise of extracellular K + upon neuronal activity is expected to depolarize the glial membrane and shut down ClC-2. Dysregulation of Cl − concentrations in the small extracellular clefts might also change extracellular pH through Cl − /HCO 3 − exchangers [9] . Cell type-specific disruption of ClC-2 will be needed to clarify whether leukodystrophy results from a loss of ClC-2 currents in OLs, astrocytes or both. Genetic evidence, however, showed that GlialCAM loss elicits leukodystrophy only in part through ClC-2. Since pathology was more severe in Clcn2 −/− / Glialcam −/− than in Clcn2 −/− mice, GlialCAM ablation has additional, ClC-2-independent pathogenic effects. The lack of GlialCAM-mediated cell adhesion may also come into play, but the low abundance of GlialCAM in myelin sheaths and the prominence of other adhesion molecules [49] makes a direct role in myelin vacuolization unlikely. Moreover, vacuolization developed after apparently normal brain and myelin development, an observation that is important in view of the report [24] that overexpression of GlialCAM in U373-MG glioblastoma cells induces glial differentiation. It seems more likely that the downregulation or mislocalization of other proteins like MLC1 may contribute, together with changes in ClC-2, to MLC pathology. Unfortunately, except for its role in leukodystrophy and its protein interaction partners, not much is known about the function of MLC1. This work has revealed important functional interactions in vivo of ClC-2, GlialCAM and MLC1 ( Table 1 ), three proteins underlying human leukodystrophies. In vitro studies had shown that the adhesion molecule GlialCAM directly interacted with either MLC1 or ClC-2, changing their subcellular localization and profoundly altering ClC-2 currents [12] . However, no effect of MLC1 on GlialCAM or ClC-2 had been described. Here we showed that in addition to GlialCAM also MLC1, but not ClC-2, is important for tethering the protein complex to specific plasma membrane domains of both astrocytes and OLs in vivo . Although GlialCAM, together with MLC1, anchors ClC-2 in both types of glia, the rectification of ClC-2 Cl − currents was only abolished in OLs. Hence, the localizing effect of GlialCAM can be dissociated from its impact on ClC-2 channel function. Reduction or change in ClC-2 currents is common to all forms of leukodystrophy studied here. Hence mutations in both GLIALCAM and MLC1 may cause leukencephalopathy in part through impaired brain ion homoeostasis. Crosses between Clcn2 −/− and Glialcam −/− mice, however, show that the loss of GlialCAM or MLC1 has additional pathogenic effects unrelated to ClC-2. The unexpected similar effects of Mlc1 and Glialcam ablation on their protein partners rationalize the undistinguishable symptomatology of the MLC1 and MLC2A forms of human leukodystrophy. Mice All animal experiments were approved and in compliance with LaGeSo, Berlin, Germany, and the Animal Care and Ethics Committee of the IDIBELL and the rules set by the Government of Cataluña, Spain. Experiments were performed with mice at different ages (indicated in figure legends), and both sexes were used interchangeably. Mlc1 −/− mice were generated by Institut Clinique de la Souris (Strasbourg, France). The targeting vector was obtained from amplification of BAC RP 24-467H19 (5′-arm) and from amplification of 129S2/SvPas genomic DNA (3′-arm). Exons 2 and 3 were flanked by loxP sites. Exon 3 contained additionally a neomycin cassette flanked by FRT sites. The targeting vector was introduced into the H129 embryonic stem (ES) cell strain by electroporation and positive clones were selected by PCR. Homologous recombination was confirmed by Southern blotting and chromosomal integrity was checked by karyotyping. Correctly targeted ES cell clones were injected into C57BL/6 blastocysts and chimeric animals were crossed to FLPrecombinase expressing ‘deleter’ mice (in C57BL/6 background) to remove the neomycin-resistant cassette. To generate Mlc1 −/− mice, Mlc1 lox/lox mice were crossed to Cre-deleter mice to remove the floxed exons 2 and 3. PCR genotyping was performed using primer sequences 5′-CTGAATCTAGATGAGTTTGGGTGGC-3′ (P1); 5′-GAAACCCTCTAATTGTAGTAAGTG-3′, 5′-GAAAACCCTCTAATTGTAGTAAGTG-3′ (P2); and 5′-GCACCACAGCACCACAACATGC-3′ (P3). Mice carrying the dominant-negative mutation G89S in exon 2 of the Gliacam ( Hepacam ) gene ( Glialcam dn/dn ) and additionally having exons 2–4 flanked by loxP sites were generated by TaconicArtemis (Cologne, Germany) and were kept in a C57Bl/6 genetic background. The targeting vector was generated from BAC clones of the C57BL/6J RPCIB-731 library. Two positive selection markers, a neomycin-resistant cassette flanked by FRT sites and a puromycin-resistant cassette flanked by F3 sites, were inserted into introns 1 and 4, respectively. The targeting vector was introduced into the C57BL/6 NTac ES cell line by electroporation and positive clones were selected by PCR, and homologous recombination was confirmed by Southern blotting. Correctly targeted ES cell clones were injected into C57BL/6 blastocysts and chimeric animals were crossed to FLPe recombinase expressing ‘deleter’ mice (in C57BL/6 background) to remove neomycin and puromycin-resistant cassettes. To generate Glialcam −/− mice, Glialcam dn/dn mice were crossed to Cre-deleter mice (in C57BL/6 background) to remove the ‘floxed’ exons 2–4. PCR genotyping was performed using primer sequences 5′-CTATTTCCTGCCATACTACCTCC-3′ (P1), 5′-TGCCTTTGCTTTCTCAGTCC-3′ (P2) and 5′-TGAGCACAGACGCAACTCC-3′ (P3). Generation of Clcn2 −/− mice has been described previously [9] . Mice expressing low levels of ClC-2 (hypomorph Clcn2 , Clcn2 hyp/hyp ) were generated unintentionally by insertion of loxP sites flanking exons 2 and 3 of Clcn2 . A 10.6-kb fragment of R1 ES cell genomic DNA containing exons 1–21 of Clcn2 were cloned into pKO Scrambler Plasmid 901 (Lexicon Genetics Inc.). A neomycin-resistant cassette flanked by loxP sites and AscI sites at both ends was inserted into the ClaI site between exons 1 and 2 in a double-blunt manner. A third loxP site and an additional EcoRV site to aid Southern blot analyses were inserted between exons 3 and 4. The targeting construct was introduced into R1 ES cells by electroporation and positive clones were selected by Southern blot analyses. Selected positive clones were then electroporated with a Cre recombinase expression construct for removal of the neomycin-resistant cassette. Clones that had the neomycin-resistant cassette removed were chosen for injection into C57BL/6 blastocysts. PCR genotyping was performed using primers 5′-TTAGGCTGGAATTTGCCCGAGAGG-3′ (P1), 5′-GAGGAGGTGAGCAAGACAAAAGGG-3′ (P2) 5′-GGCAAAGGCTGGCGAGGTAACTTC-3′ (P3) and 5′-AGGGAAGGCAAGGCTAGAGAAGGC-3′ (P4). Clcn2 −/− , Mlc1 −/− and Clcn2 hyp/hyp mice were in a C57BL/6-129/Svj mixed genetic background, while Glialcam −/− and Glialcam dn/dn were in a C57BL/6 background. For some electrophysiological measurements mice were crossed to a transgenic line expressing enhanced green fluorescence protein under the control of the human GFAP promotor [22] (FVB/N background), resulting in enhanced green fluorescence protein expression in astrocytes. Generation of antibodies Antibodies against mouse ClC-2 were raised in rabbits against two peptide sequences of different length corresponding to the extreme C terminus: (C)WGPRSRHGLPREGTPSDSDDK S Q (used for western blotting) and (C)HGLPREGTPSDSDDK S Q (by Biogenes, Berlin, Germany; used for immunofluorescence staining). A cysteine in the native protein sequence was replaced by the highlighted serine to prevent coupling of this residue to the carrier protein. GlialCAM-specific antibodies used for western blots were raised in rabbits to peptide (C)LKDKDSSEPDENPATEPR, and those used for immunostainings were raised in guinea pigs to peptide (C)AGVQRIREQDESGQVEISA. Both peptide sequences correspond to non-overlapping parts of the intracellular C-terminal region of mouse GlialCAM. Antibodies recognizing the amino terminus of mouse MLC1 (used for immunostaining) were raised in rabbits and guinea pigs against peptide TREGQFREELGYDRM(C) [20] . Antibodies to the MLC1 C terminus (used for western blotting) were raised in rabbits against peptide CPQERPAGEVVRGPLKEFDK. Generation of antibodies was performed by Pineda Antibody Services (Berlin, Germany), unless indicated otherwise. ‘(C)’ indicates cysteines not included in native protein sequence that were added to facilitate coupling to carrier protein. Antibodies were affinity purified from serum using the immunizing peptide. Western blot analyses For western blot analyses, membrane fractions were isolated from mouse tissue. To this end, tissue homogenate was prepared in 20 mM Tris–HCl pH 7.4, 140 mM NaCl, 2 mm EDTA with protease inhibitors (4 mM Pefabloc and Complete EDTA-free protease inhibitor cocktail, Roche) using a glass Dounce homogenizer and cleared by centrifugation for 10 min at 1,000 g . Membrane fractions were pelleted from the cleared homogenate by ultracentrifugation for 30 min at 270,000 g , and the pellet was resuspended by sonification in 50 mM Tris pH 6.8, 140 mM NaCl, 2 mM EDTA with protease inhibitors. Equal amounts of protein were separated by SDS–polyacrylamide gel electrophoresis and blotted onto nitrocellulose. Blots were reprobed with mouse anti-β-actin (Clone AC-74, Sigma A2228, 1:5,000) as a loading control. Immunohistochemistry Deeply anaesthetized mice were perfused with 1% paraformaldehyde (PFA) in PBS and 6 μm sagittal cryosections were prepared from brains. Sections were postfixed with 1% PFA/PBS for 10 min, permeabilized with 0.2% Triton-X100 in PBS and blocked with 3% BSA in PBS. Antibodies were diluted in blocking buffer. Incubation with primary antibody (see below for dilution) was performed at 4 °C overnight, incubation with secondary antibodies (1:1,000) coupled to Alexa fluorophores (Molecular Probes) was carried out for 1 h at room temperature. Nuclei were stained with 4',6-diamidino-2-phenylindole (Sigma). In addition to the self-generated primary antibodies described above, the following commercial antibodies were used: mouse anti-GFAP (clone G-A-5, Sigma G3893, 1:1,000), mouse anti-S100β (clone SH-B1, Sigma S2532, 1:1,000), mouse anti-APC (clone CC1, Merck Millipore OP80, 1:200) and rat anti-heparan-sulphate-proteoglycan (perlecan, clone A7L6, Merck Millipore MAB1948P, 1:2,000) and goat anti-aquaporin-4 (Santa Cruz sc-9888, 1:50). The rabbit anti-Kir4.1 (used here at a dilution of 1:100) was kindly provided by S Takeuchi [50] . Images were acquired using an LSM510 confocal microscope and ZEN software (Zeiss). Histology For histological analyses of brains and eyes, mice were perfused with 4% PFA/PBS and organs were postfixed overnight. Haematoxylin–eosin staining was performed on 6 μm paraffin sections of brains and eyes. Electron microscopy For ultrastructural studies, deeply anaesthetized mice were transcardially perfused with 4% paraformaldeyhde (PFA) and 2.5% glutaraldehyde in 0.1 M PB (pH 7.4). The brains were removed and cut vertically into two halves. The brain samples were postfixed in the same fixative overnight at 4 °C. Brains were cut into 150 μm sagittal sections of the cerebellum with a Leica vibratome. Cerebellum sections were cut into 1 mm 3 fragments. They were rinsed with 0.1 M PB (pH 7.4) and postfixed with 2% aqueous osmium tetroxide and 1.5% potassium hexacyanoferrate (K3[Fe(CN)6]) for 30 min. After rinsing with 50% ethanol, sections were stained en bloc with 1% uranylacetate for 1 h in 70% ethanol. Fragments were dehydrated in graded ethanol, followed by infiltration of propylene oxide and embedding in Epon (Electron Microscopic Sciences, Hatfield, PA, USA). Ultrathin sections (60 nm) were prepared with a Reichert Ultracut S, stained in 5% uranylacetate and 0.4% lead citrate ((C6H5O7)2Pb3). Stained ultrathin sections were examined with a Zeiss 902 at 80 kV and a Fei Tecnai G F20 at 200 kV. Photographs were taken with a Megaview 3 Camera and a Gatan Ultrascan 1000 Camera. Two mice per genotype were examined, with more than 10 ultrathin sections each and that displayed consistent results. Molecular biology For quantitative real-time PCR, total RNA was isolated from the cerebellum of 11–18-week-old mice using the RNeasy lipid tissue mini kit with on-column DNase digestion (Qiagen). Complementary DNA was synthesized from 1 μg of RNA using Superscript II reverse transcriptase (Invitrogen). PCR reactions were prepared using Power Sybr Green PCR Master Mix (Applied Biosciences) and ran in triplicates in a StepOnePlus Real-Time PCR System with StepOne Software (Applied Biosystems) to monitor amplification and melting curves. Relative expression of mutant mice compared with WT siblings was calculated using the ΔΔCT method and β-actin as an internal control. The following primers were used: 5′-GACCGCCTAAAATCAGAAGCA-3′ and 5′-TGGCTCTGTAGCAGGGTTTT-3′ for Glialcam ; 5′-TCAGTGCGATTCCCAACTTTCA-3′ and 5′-GGACCGGGCCGAAATGAT-3′ for Mlc1 . Primer sequences for Clcn2 : 5′-CAGTGACTGCAAAATCGACCC-3′ and 5′-CATAAGCATGGTCCACTCCCA-3′ and for β-actin: 5′-TGTGATGGTGGGAATGGGTCAGAA-3′ and 5′-TGTGGTGCCAGATCTTCTCCATGT-3′ as described previously [8] , [51] . Missplicing in Clcn2 hyp/hyp was detected by semiquantitative reverse transcription–PCR. Total RNA was isolated from brain using Trizol reagent (Invitrogen) and cDNA synthesis was performed as described above. Subsequently, PCR was performed using the following primer sequences: 5′-ATGGCGGCTGCAACGGCTG-3′ and 5′-AGGTTAGCCCAATGACCTTAGC-3′. Expression constructs for mouse Glialcam and Mlc1 were generated by PCR using full-length cDNA clones (SourceBioScience) as templates. Where applicable, C-terminal haemagglutinin (HA) tags were added by PCR and constructs were cloned into the pcDNA3.1 mammalian expression vector (Invitrogen). The cDNAs for rat Clcn2 and human Glialcam were cloned in the pFROG vector for expression with the mammalian CMV promoter. Cell culture/transfection HeLa cells (DSMZ, Germany, ACC 57, lot 17) were transfected with Clcn2 , Glialcam or Mlc1 expression constructs using polyethylenimine. One day post transfection, cells were split and seeded onto coverslips. Three days after transfection, cells were fixed with 4% PFA/PBS, permeabilized with 0.2% Triton-X100/PBS and subjected to antibody staining as described for immunohistochemistry on tissue sections. Electrophysiological analysis of glial cells in brain slices Unless specified, concentrations are in mM and all solutions for incubating slices were constantly oxygenated with carbogen (5% CO 2 in O 2 ). Mice (3–4 weeks old of both gender) were deeply anaesthetized and either 200 μm sagittal sections for BG or 150 μm coronal sections for corpus callosum OLs were prepared using a vibrating microtome (Leica VT1200S, Germany) in ‘low Ca 2+ ’ artificial cerebrospinal fluid (aCSF) containing: 134 NaCl, 2.5 KCl, 10 glucose, 26 NaHCO 3 , 1.25 K 2 HPO 4 , 1.3 MgCl 2 , and 0.2 CaCl 2 and adjusted to pH 7.4 with NaOH and to 325±5 mOsm kg −1 . Sagittal slices were allowed to recover in standard aCSF (2 CaCl 2 ) for at least 45 min at room temperature. Coronal slices, following sectioning, were first heated at 37 °C for 30 min in standard aCSF before transferring to room temperature. Measurements were performed at room temperature. Slices were adhered to poly- L -lysine-coated coverslips and transferred to a recording chamber (Luigs & Neumann, Germany) with constant perfusion of aCSF (1–2 ml min −1 ) and mounted to an upright microscope equipped with a × 60 water immersion objective and both differential interference contrast and fluorescence optics (Olympus BX51WI). Patch pipettes were fabricated from glass capillaries (World Precision Instruments PG52151-4, USA; DMZ Universal Puller, Germany) and filled with an intracellular solution containing: 140 CsCl, 1 MgCl 2 , 10 HEPES, 5 EGTA, 0.2 disodium carbenoxolone (Sigma-Aldrich) and adjusted to pH 7.3 with CsOH and to 290 mOsm kg −1 . Either 0.5 mg ml −1 Alexa Fluor 488 (Life Technologies A10436) or 2 mg ml −1 biocytin (Sigma B4261) was added to the patch pipette to confirm cell identity during the recording or following slice fixation for post hoc analysis, respectively. Ag-AgCl wires were used for recording and reference electrodes. Using a computer-controlled microelectrode amplifier (Multiclamp 700B) and acquisition software (Clampex 10.3, Molecular Devices, USA), patch pipettes typically registered resistances of 5–7 MΩ with a small voltage pulse. For patch clamping of BG and OLs in the tight seal configuration (>1 GΩ), small somata adjacent to the larger Purkinje cells were selected, and small somata typically grouped in a row parallel to fibres in white matter tracts were selected, respectively. On acquisition of the conventional whole-cell configuration, large voltage-independent currents were seen in both BG and OLs on short voltage pulses from +40 to −100 mV from a holding potential of −10 mV. Morphologically, BG typically had two or three thin processes radiating across the molecular layer and terminating in the pia. OLs typically had processes that were sparsely branched and were orientated in parallel with myelinated fibres. To isolate ClC-2 currents, slices were perfused with a Na + - and K + -free extracellular solution containing: 117 NMDG-Cl, 23 NMDG-HCO 3 , 5 CsCl, 1.3 MgCl 2 , 9 glucose, 2 CaCl 2 , 0.2 Na 2 -carbenoxolone and adjusted to pH 7.3 with CsOH and 295±5 mOsm kg −1 . Typically, at least 10–15 min were needed before the membrane conductance stabilized on perfusion with the NMDG-Cl bath solution. To elicit ClC-2 currents, voltage steps from +40 to up to −120 mV from a holding potential of −10 mV were used. A final 1 s voltage step at +40 mV was applied before returning to the holding potential. Signals were digitized at 10 KHz, filtered at 2 kHz and stored for off-line analysis. Using the standard membrane test function in Clampex software, membrane capacitance and resistances were obtained online at the end of the experiment using a small 5 mV pulse from a holding potential of −10 mV. In some experiments, slices were perfused with either a hypotonic diluted NMDG-Cl solution (80%) to 235±5 mOsm kg −1 , or a hypertonic NMDG-Cl with sucrose added to 325±5 mOsm kg −1 . Averaging, normalizing and subtracting trace profiles were done off-line using ClampFit 10.3 (Molecular Devices). Current profiles were acquired using the same voltage pulse protocol (1.5 s steps from +40 to −120 mV including a 1-s tail current at +40 mV before returning back to the holding potential of −10 mV). Currents from each cell were averaged by genotype to obtain an average current (I) profile. In other analyses, the average I profile from each genotype was divided (‘Arithmetic tool’) by its average capacitance (C) to obtain the average current density (I/C) profile. For trace subtraction, either I or I/C trace profiles from Clcn2 −/− mice were subtracted (‘Arithmetic tool’) from the respective I or I/C trace profiles from WT, Glialcam −/− , Mlc1 −/− , Glialcam dn/dn or Glialcam +/− animals to examine the ClC-2-specific I or I/C trace profiles in the different mouse models. Processing of biocytin-filled cells in brain slices Following patch clamp experiments, slices were fixed in 4% PFA (in 1 × PBS) overnight at 4 °C. Slices were washed in wash buffer containing 0.1 M PB pH 7.4 and 0.25% Triton-X100. Slices were blocked in wash buffer containing 5% normal goat serum for 2 h at room temperature. For secondary detection, Alexa Fluor 555 Streptavidin (Life Technologies) was added to the slices at a 1:500 dilution for overnight incubation at 4 °C. Slices were washed and mounted on gelatinized slides with Fluoromount G (SouthernBiotech). Images were acquired with a confocal microscope (Zeiss LSM 510). Patch clamp measurements in HEK cells HEK293 cells were transfected in 12-well plates at ~50% confluency with either 0.5 μg of plasmid encoding rat ClC-2 or 0.25 μg of plasmid encoding rat ClC-2 and 0.25 μg of plasmid encoding human Glialcam. All cells were co-transfected with a reporter plasmid expressing GFP. Using a microelectrode amplifier (Multiclamp 700B) with acquisition software (Clampex 10.3; Molecular Devices, USA), whole-cell currents were measured by patch clamp analysis 2 days after transfection. When filled with an intracellular solution containing (in mM): 140 CsCl, 1 MgCl 2 , 10 HEPES and 5 EGTA adjusted to pH 7.3 and to 290± mOsm kg −1 , patch pipettes registered resistances of 4–5 MΩ. The bath solution was composed of (in mM): 140 NaCl, 2 MgSO 4 , 2 CaCl 2 , 10 HEPES, 22 sucrose and adjusted to pH 7.4 with NaOH and to 325±5 mOsm kg −1 with sucrose. ClC-2 currents were elicited with 1 s voltage pulses from +40 to −120 mV and a final voltage pulse at +40 mV before returning back to the holding potential of −10 mV. Individual cells were first measured in normal bath solution and again following superfusion of bath solution containing 200 μM disodium carbenoxolone. Signals were digitized at 10 KHz, filtered at 2 kHz and stored for off-line analysis using ClampFit software. Statistics Statistical significance was assessed between two groups using the non-parametric Mann–Whitney test (Prism, GraphPad Software, USA). How to cite this article: Hoegg-Beiler, M. B. et al. Disrupting MLC1 and GlialCAM and ClC-2 interactions in leukodystrophy entails glial chloride channel dysfunction. Nat. Commun. 5:3475 doi: 10.1038/ncomms4475 (2014).